Dissociation of Bak α1 helix from the core and latch domains is required for apoptosis During apoptosis, Bak permeabilizes mitochondria after undergoing major conformational changes, including poorly defined N-terminal changes. Here, we characterize those changes using 11 antibodies that were epitope mapped using peptide arrays and mutagenesis. After Bak activation by Bid, epitopes throughout the α1 helix are exposed indicating complete dissociation of α1 from α2 in the core and from α6–α8 in the latch. Moreover, disulfide tethering of α1 to α2 or α6 blocks cytochrome c release, suggesting that α1 dissociation is required for further conformational changes during apoptosis. Assaying epitope exposure when α1 is tethered shows that Bid triggers α2 movement, followed by α1 dissociation. However, α2 reaches its final position only after α1 dissociates from the latch. Thus, α1 dissociation is a key step in unfolding Bak into three major components, the N terminus, the core (α2–α5) and the latch (α6–α8). Bak and Bax are pro-apoptotic members of the Bcl-2 protein family that controls apoptosis [1] , [2] . In healthy cells, Bak and Bax exist in inert conformations in which their hydrophobic α5 helices are surrounded by seven or eight amphipathic helices [3] , [4] . A carboxy (C)-terminal helix, α9, anchors Bak constitutively in the mitochondrial outer membrane (MOM) [5] , [6] , whereas in Bax, the α9 helix is initially sequestered in the hydrophobic surface groove, rendering Bax largely cytosolic [4] , [7] . When cells experience sufficient stress, the BH3-only class of Bcl-2 family proteins cause Bak and Bax to undergo a series of conformation changes—collectively referred to as ‘activation’—that culminate in dimerization, leading to pore formation in the MOM [8] , [9] , [10] . Pore formation releases cytochrome c into the cytosol to initiate caspase activation and dismantle the cell [11] . Bak activation is triggered by binding of BH3-only proteins (for example, Bid or Bim) to a hydrophobic groove on the Bak surface [11] , [12] . Two major consequences are exposure of the BH3 domain in α2 (ref. 9 ) and exposure of epitopes in the Bak amino (N) terminus [10] , [13] . The N terminus comprises a semi-structured N-segment (aa1–23) [14] and the α1 helix (aa24–50) containing the BH4 domain [15] . Similar conformation changes occur in Bax during its activation [16] , [17] , [18] . Another key conformation change identified in Bak and Bax is separation of the latch (α6–α8) from the core (α2–α5) [19] , [20] . After these large changes in conformation, the proteins form BH3:groove dimers and make significant contact with the outer membrane surface [9] , [16] , [19] , [21] , [22] . Elucidating the structures of the fully activated forms of Bak and Bax will provide insight into how these proteins self-associate to form the apoptotic pore. However, the Bak N-terminal epitopes exposed by activation are poorly mapped so it remains unclear whether some or all elements of the N-termini re-position during activation, or whether they are exposed by re-positioning of other elements, for example, the α6–α8 latch domain [19] or by dissociation of Bak from other proteins such as VDAC2 (refs 10 , 23 ). To gain insight into the molecular changes occurring at the Bak N terminus during apoptosis, we mapped the epitopes of 11 anti-Bak antibodies using peptide arrays and mutagenesis. We also developed a novel fluorescence-activated cell sorting (FACS) protocol for measuring epitope exposure after disulfide tethering, which allowed us to examine the sequence of Bak conformation changes during activation. Herein, we show that N-terminal epitopes of Bak are mostly linear, and that many are located within the α1 helix including two that overlap with the BH4 domain of Bak. All epitopes within α1 and the N-segment are conformation specific as their exposure increases upon Bak activation. Intramolecular tethering demonstrated that separation of α1 and α6, and of both from the core, is required for pore formation. In addition, dissociation of α1 from α2 is required for BH3:groove dimer formation. Thus dissociation of α1 from both the core and latch domains is a key event in the activation of Bak. Most Bak antibodies have linear epitopes To investigate Bak N-terminal conformation change during apoptosis, we compared the binding properties of 11 anti-Bak antibodies. 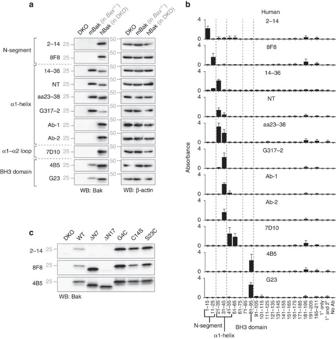Figure 1: Mapping N-terminal epitopes of Bak. (a) Bak antibodies recognize linear epitopes in human Bak, but only a subset recognize mouse Bak. Lysates from MEF expressing no Bak (Bax−/−Bak−/−(DKO)), mouse Bak (Bax−/−) or WT human Bak (in DKO) were analysed by western blot using the indicated antibodies. Blots were re-probed with β-actin to compare loading. Data are representative of two independent experiments. (b) Most Bak epitopes map to peptides from the N terminus. Histograms showing immunoreactivity of Bak antibodies towards biotinylated 15-mer hBak peptides, as determined by enzyme-linked immunosorbent assay. X axis labels indicate residue number or control reaction conditions. Data are mean and s.d. of three independent experiments. (c) The epitopes of antibodies binding in the Bak N-segment are distinct. The 2–14 and 8F8, which bound to peptides corresponding to N-segment residues inb, were tested by western blot for their ability to bind N-terminally truncated or single residue mutants of hBak (as indicated) expressed in DKO MEF. On the basis of loss of signal, residues 1–7 are required for the 2–14 antibody to bind Bak, whereas residues 8–17 are required for the 8F8 antibody to bind Bak (as also shown in ref.14). Binding by 4B5 is shown as a reference for expression levels of various mutants, since its epitope in the BH3 domain is C-terminal to the N-segment9. Data are representative of two independent experiments. Table 1 lists known characteristics of the antibodies, together with the key residues involved in their epitopes, as determined below. Table 1 Features of Bak antibodies. Full size table Antibodies were first tested by SDS–polyacrylamide gel electrophoresis (SDS–PAGE) and western blotting to determine if their epitopes were linear (also called continuous or sequential epitopes) or assembled (also called discontinuous or conformational epitopes) [24] . As all antibodies recognized human Bak after SDS–PAGE ( Fig. 1a ), each epitope was linear. Figure 1: Mapping N-terminal epitopes of Bak. ( a ) Bak antibodies recognize linear epitopes in human Bak, but only a subset recognize mouse Bak. Lysates from MEF expressing no Bak ( Bax −/− Bak −/− (DKO)), mouse Bak ( Bax −/− ) or WT human Bak (in DKO) were analysed by western blot using the indicated antibodies. Blots were re-probed with β-actin to compare loading. Data are representative of two independent experiments. ( b ) Most Bak epitopes map to peptides from the N terminus. Histograms showing immunoreactivity of Bak antibodies towards biotinylated 15-mer hBak peptides, as determined by enzyme-linked immunosorbent assay. X axis labels indicate residue number or control reaction conditions. Data are mean and s.d. of three independent experiments. ( c ) The epitopes of antibodies binding in the Bak N-segment are distinct. The 2–14 and 8F8, which bound to peptides corresponding to N-segment residues in b , were tested by western blot for their ability to bind N-terminally truncated or single residue mutants of hBak (as indicated) expressed in DKO MEF. On the basis of loss of signal, residues 1–7 are required for the 2–14 antibody to bind Bak, whereas residues 8–17 are required for the 8F8 antibody to bind Bak (as also shown in ref. 14 ). Binding by 4B5 is shown as a reference for expression levels of various mutants, since its epitope in the BH3 domain is C-terminal to the N-segment [9] . Data are representative of two independent experiments. Full size image To gain insight into the possible location of the epitopes, we also tested each antibody for its ability to bind mouse Bak, since the mouse Bak protein sequence is 77% similar to human Bak and the antibodies were unlikely to bind in regions of sequence divergence. Six antibodies (14–36, NT, aa23–38, G317-2, 4B5 and G23) also recognized mouse Bak ( Fig. 1a ). For three of these antibodies (14–36, NT and aa23–38), the immunogen contained a stretch of residues (26–36) conserved in mouse and human Bak ( Table 1 ). Another two antibodies (4B5 and G23) had previously been mapped to a conserved region [9] . Epitopes map to various sites in the Bak N terminus As the Bak epitopes were linear, further mapping was performed using peptide arrays. When applied to an array of overlapping 15-mer peptides from human Bak, all antibodies bound to at least one peptide ( Fig. 1b ). When applied to a similar array of mouse Bak peptides, the six antibodies that bound mouse Bak on western blots ( Fig. 1a ) also recognized at least one peptide ( Supplementary Fig. 1 ). Epitope mapping by peptide array was consistent with the immunogen sequence and previous mapping data ( Table 1 ), and together the panel of antibodies recognized at least five distinct epitopes in the N terminus ( Fig. 1b ). Note, the N-segment positions of the 2–14 and 8F8 epitopes suggested by the array were confirmed by western blotting of N-terminally truncated Bak ( Fig. 1c ). As seven antibodies (14–36, NT, a23–38, G317-2, Ab-1, Ab-2, 7D10) bound peptides containing α1 residues, we focused on mapping their epitopes further and designed an array of 8-mers with only a single residue offset to define the minimal set of residues required for their binding. As expected, due to their polyclonal nature the three peptide-derived antibodies (14–36, NT and aa23–38) produced complex binding patterns for this array ( Supplementary Fig. 2 ), while the monoclonal antibodies (G317-2, Ab-1, Ab-2 and 7D10) produced simple binding patterns. G317-2 bound four peptides ( Fig. 2a ) refining its epitope to 32 EEVFR 36 , and suggesting that E32 and R36 are particularly important for its binding. Ab-1 and Ab-2 bound predominantly to the same peptide 38 YVFYRHQQ 45 , suggesting their epitopes are very similar. The 7D10 epitope begins after α1, with 51 GVAAP 55 the minimal set of residues required for binding. Thus, peptide arrays of increasing resolution defined the minimal linear epitopes of several antibodies to the Bak N terminus. 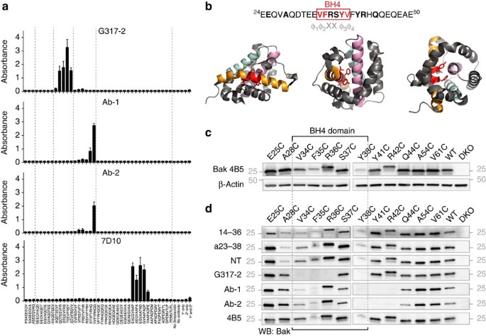Figure 2: Epitopes in α1 and residues of α1 important for Bak stability. (a) Precise positioning of the G317-2, Ab-1, Ab-2 and 7D10 epitopes. Histograms showing immunoreactivity of Bak antibodies towards biotinylated 8-mer peptides that collectively span residues 20–65 of human Bak. X axis labels indicate peptide sequence or control reaction conditions. Data are mean and s.d. of three independent experiments. (b) Diagrams showing the position of the BH4 domain15in the Bak α1 sequence and structure of inactive Bak (PDB: 2IMS, ref.3). Residues in bold were mutagenized for experiments illustrated in (c) and (d). Three different orientations of the structure are shown. Note the hydrophobic side-chains of the BH4 domain (red) within α1 (yellow) point towards α5 (pink) and α6 (cyan) residues in the core of Bak. (c) Hydrophobic residues in the BH4 domain are important for Bak function. Lysates from DKO MEF expressing Bak α1 cysteine mutants were analysed by western blot. Y38C, F35C and, to a lesser extent, V34C exhibited consistently weaker signals than other α1 mutants. E25C migrates a little faster and R36C and R42C slightly slower than WT hBak, due to their cysteine substitutions changing the overall net charge of Bak40. Blots were re-probed with β-actin to compare loading. Data are representative of two independent experiments. (d) Three sets of Bak α1 residues (Α28, V34-R36 and S37-Q44) are important for antibody binding. The ability of antibodies (indicated on the left) to bind Bak α1 cysteine mutants (indicated above) was compared by western blotting. Lysates from DKO MEF expressing no Bak, WT Bak or mutations C-terminal to α1 (A54C, V61C) were included as negative and positive controls. Data are representative of three independent experiments. Figure 2: Epitopes in α1 and residues of α1 important for Bak stability. ( a ) Precise positioning of the G317-2, Ab-1, Ab-2 and 7D10 epitopes. Histograms showing immunoreactivity of Bak antibodies towards biotinylated 8-mer peptides that collectively span residues 20–65 of human Bak. X axis labels indicate peptide sequence or control reaction conditions. Data are mean and s.d. of three independent experiments. ( b ) Diagrams showing the position of the BH4 domain [15] in the Bak α1 sequence and structure of inactive Bak (PDB: 2IMS, ref. 3 ). Residues in bold were mutagenized for experiments illustrated in ( c ) and ( d ). Three different orientations of the structure are shown. Note the hydrophobic side-chains of the BH4 domain (red) within α1 (yellow) point towards α5 (pink) and α6 (cyan) residues in the core of Bak. ( c ) Hydrophobic residues in the BH4 domain are important for Bak function. Lysates from DKO MEF expressing Bak α1 cysteine mutants were analysed by western blot. Y38C, F35C and, to a lesser extent, V34C exhibited consistently weaker signals than other α1 mutants. E25C migrates a little faster and R36C and R42C slightly slower than WT hBak, due to their cysteine substitutions changing the overall net charge of Bak [40] . Blots were re-probed with β-actin to compare loading. Data are representative of two independent experiments. ( d ) Three sets of Bak α1 residues (Α28, V34-R36 and S37-Q44) are important for antibody binding. The ability of antibodies (indicated on the left) to bind Bak α1 cysteine mutants (indicated above) was compared by western blotting. Lysates from DKO MEF expressing no Bak, WT Bak or mutations C-terminal to α1 (A54C, V61C) were included as negative and positive controls. Data are representative of three independent experiments. Full size image The BH4 domain in α1 is critical for Bak stability To analyse the role of α1 in Bak function, we utilized 10 variants of Bak in which residues (E25, Α28, V34, F35, R36, S37, Y38, Y41, R42, Q44) were substituted with cysteine ( Fig. 2b,c ). After stable expression in Bak −/− Bax −/− MEF, most variants were present at levels similar to that of wild-type human Bak ( Fig. 2c ), indicating that cysteine substitution had not significantly altered protein expression or stability. The exceptions were three variants (V34C, F35C, Y38C) that were present at only low levels ( Fig. 2c ). Notably, these residues lie in the BH4 domain of Bak ( Fig. 2b ), the sequence motif present in all multidomain members of the Bcl-2 family, including viral prosurvival proteins [15] . The destabilizing effect of cysteine substitution within the BH4 domain is consistent with the high conservation of this motif [15] and with observations that truncating Bak α1 results in low protein levels after retroviral expression [14] . The BH4 domain contributes to the G317-2 and Ab-1 epitopes The cysteine-substituted Bak variants were also used to test whether the residues within α1 epitopes were required for antibody binding ( Fig. 2d ). Among the polyclonal antibodies, both a23–38 and NT bound weakly to A28C ( Fig. 2d ), indicating that dominant epitopes among their collections of immunoglobulins overlap and that most depend on A28. The epitopes of 14–36 were also sensitive to mutation of A28 ( Fig. 2d ). Notably, each of the epitopes for the monoclonal antibodies relied on at least some residues within the BH4 domain ( 34 VFRSYV 39 ). G317-2 failed to bind V34C, F35C and R36C, consistent with its epitope being at EEVFR. Ab-1 and Ab-2 failed to bind Y38C, Y41C and R42C, consistent with their epitope being within YVFYRHQQ, and with a recent report that Y38 is critical for Ab-1 binding [25] . Thus, the anti-Bak antibodies tested bound to three distinct sites (residues 28, 34–36 and 37–44) along α1. ‘N-terminal exposure’ involves complete dissociation of α1 Antibodies generated to the Bak N terminus have often been used to monitor Bak conformation change (activation) during apoptosis [10] , [13] , [14] . In particular, Ab-1 has been widely used as a ‘conformation-specific’ antibody to report ‘N-terminal exposure’ of Bak during apoptosis [10] . Based on our mapping of the Ab-1 epitope, two residues (Y38 and R42) required for Ab-1 binding are buried in the structure of non-activated Bak ( Supplementary Fig. 3 ), arguing that this central region of α1 must become exposed during apoptosis. A similar argument holds for the start of α1, as the NT antibody recognizes only activated Bak [13] and its epitope includes both Α28 ( Fig. 2d ) and T31 [25] , which are also buried in non-activated Bak ( Supplementary Fig. 3 ). The N-segment also undergoes conformation change, as 8F8 binds preferentially to activated Bak [14] . Thus, based on literature reports of three ‘conformation-specific’ antibodies (8F8, NT, Ab-1) and epitope mapping of those antibodies, at least three distinct sites (11–17, 28–31 and 38–45) in the N terminus become exposed during Bak activation. To further examine Bak N-terminal exposure during apoptosis, five additional N-terminal antibodies were tested for immunoprecipitation of Bak before and after activation by Bid ( Fig. 3 ). Three cell lines were used to compare recognition of endogenous mouse and human Bak with exogenous human Bak. All five antibodies bound to Bak more efficiently after its activation ( Fig. 3 ). The 14–36 and G317-2 antibodies were most efficient in the conditions used ( Fig. 3 , compare bound and unbound fractions). The specificity of these additional five antibodies for an active conformation thus confirms that the entire N terminus (that is, the N-segment and α1) dissociates from the remainder of the protein during Bak activation. Furthermore, when monitored by Ab-1 or G317-2 epitope exposure, this conformation change may be considered ‘BH4 exposure’, much as 4B5 or G23 epitope exposure signifies ‘BH3 exposure’. 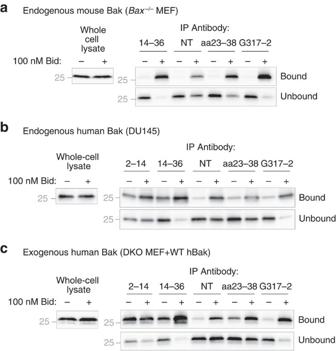Figure 3: All Bak N-terminal epitopes are exposed during activation. Membrane fractions from cells expressing endogenous mouse or human Bak (a,brespectively) or exogenous human Bak (c) were incubated (30 min, 30 °C) with (+) or without (−) Bid, solubilized with digitonin, and incubated with the Bak antibodies shown. Bak in immunoprecipitates and whole-cell lysate or unbound controls was detected by western blot using the 4B5 antibody. Data are representative of at least two independent experiments. Figure 3: All Bak N-terminal epitopes are exposed during activation. Membrane fractions from cells expressing endogenous mouse or human Bak ( a , b respectively) or exogenous human Bak ( c ) were incubated (30 min, 30 °C) with (+) or without (−) Bid, solubilized with digitonin, and incubated with the Bak antibodies shown. Bak in immunoprecipitates and whole-cell lysate or unbound controls was detected by western blot using the 4B5 antibody. Data are representative of at least two independent experiments. Full size image Dissociation of α1 from α6 is required for pore formation To better understand how Bak unfolds during activation, we examined whether BH4 exposure occurs before or after BH3 exposure. This was done by disulfide tethering the N terminus to the remainder of Bak at three positions ( Fig. 4a ). One tether (WT) utilized the native cysteines in human Bak, C14 in the N-segment and C166 in the α6–α7 loop. Two other tethers (Y41C:A79C and A28C:L163C) involved cysteine substitutions at the relevant positions in cysteine-less human Bak (C14S/C166S). Each tether was induced with high efficiency following addition of the oxidizing agent copper phenanthroline (CuPhe), as indicated by faster migration of Bak during non-reducing SDS–PAGE ( Fig. 4b ). The mutations did not alter Bak function as indicated by cytochrome c in response to Bid ( Fig. 4c ). However, in contrast to C14S/C166S Bak, when WT or cysteine double mutant Bak was incubated with CuPhe to induce tethers, cytochrome c release no longer occurred in response to Bid, Bim BH3 peptide or heat ( Fig. 4c ). These data support a recent report that tethering WT Bak blocks pore formation in response to heat [25] , and defines α1 dissociation as required for Bak pore formation. 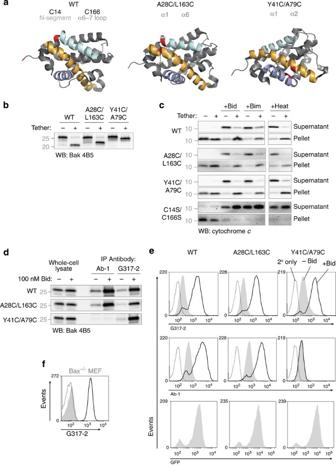Figure 4: N-terminal tethers and G317-2 detection of Bak activation by intracellular FACS. (a) Position of residues (red) in the inactive Bak structure (PDB: 2IMS, ref.3) that can be cross-linked with CuPhe to generate tethers; α1 is yellow, α6 is cyan and α2 is lilac. As the structure was derived using truncated Bak3, for WT Bak the most N-terminal residue present (S21) is marked red as a surrogate for C14. (b) Tethers were efficiently induced by CuPhe cross-linking of cysteines in non-activated Bak. DKO MEF were incubated with (+) or without (−) 200 μM CuPhe for at least 5 min, on ice. Tethered Bak appears as a faster migrating fragment after non-reducing SDS–PAGE. Differences in migration between samples reflect the positions of the tethers. Data are representative of at least three independent experiments. (c) Bak mutants are functional and all tethers block cytochromecrelease in response to apoptotic stimuli. After inducing tethers (as inb), membrane fractions were incubated with or without either 100 nM Bid, 10 μM Bim peptide or heat (44 °C). Data are representative of three independent experiments. (d) G317-2, but not Ab-1, can bind to activated Y41CA79C Bak. Membrane fractions from DKO MEF expressing hBak were treated as inFig. 3. Data are representative of three independent experiments. (e) G317-2 can substitute for Ab-1 in intracellular FACS assays for Bak activation. Permeabilized DKO MEF were treated with (solid line) or without (filled histograms) 100 nM Bid and incubated with Ab-1 or G317-2. Dotted lines show signals for cells incubated without primary antibody. FACS plots of GFP levels indicate the proportion of cells expressing Bak. The G317-2 profiles of treated cells closely match GFP levels, indicating all cells expressing Bak responded to Bid. (f) Mouse Bak activation can be measured by intracellular FACS using G317-2.Bax−/−MEF were treated as in (e). Figure 4: N-terminal tethers and G317-2 detection of Bak activation by intracellular FACS. ( a ) Position of residues (red) in the inactive Bak structure (PDB: 2IMS, ref. 3 ) that can be cross-linked with CuPhe to generate tethers; α1 is yellow, α6 is cyan and α2 is lilac. As the structure was derived using truncated Bak [3] , for WT Bak the most N-terminal residue present (S21) is marked red as a surrogate for C14. ( b ) Tethers were efficiently induced by CuPhe cross-linking of cysteines in non-activated Bak. DKO MEF were incubated with (+) or without (−) 200 μM CuPhe for at least 5 min, on ice. Tethered Bak appears as a faster migrating fragment after non-reducing SDS–PAGE. Differences in migration between samples reflect the positions of the tethers. Data are representative of at least three independent experiments. ( c ) Bak mutants are functional and all tethers block cytochrome c release in response to apoptotic stimuli. After inducing tethers (as in b ), membrane fractions were incubated with or without either 100 nM Bid, 10 μM Bim peptide or heat (44 °C). Data are representative of three independent experiments. ( d ) G317-2, but not Ab-1, can bind to activated Y41CA79C Bak. Membrane fractions from DKO MEF expressing hBak were treated as in Fig. 3 . Data are representative of three independent experiments. ( e ) G317-2 can substitute for Ab-1 in intracellular FACS assays for Bak activation. Permeabilized DKO MEF were treated with (solid line) or without (filled histograms) 100 nM Bid and incubated with Ab-1 or G317-2. Dotted lines show signals for cells incubated without primary antibody. FACS plots of GFP levels indicate the proportion of cells expressing Bak. The G317-2 profiles of treated cells closely match GFP levels, indicating all cells expressing Bak responded to Bid. ( f ) Mouse Bak activation can be measured by intracellular FACS using G317-2. Bax − / − MEF were treated as in ( e ). Full size image To assess which Bak conformation changes were hindered by these tethers, epitope exposure was quantified by flow cytometry. While Ab-1 is commonly used for flow cytometry of Bak, the Y41C substitution disrupted Ab-1 binding ( Fig. 4d,e ). Instead, we used G317-2, which only recognizes activated Bak ( Figs 3 and 4d ), and whose epitope also overlaps with the BH4 domain ( Fig. 2d ). After activation by Bid, the expected binding of G317-2 to all human Bak variants ( Fig. 4e ), as well as mouse Bak ( Fig. 4f ), was readily detectable by FACS. Thus, G317-2 is a particularly useful alternative to the Ab-1 antibody as it efficiently recognized activated forms of both human and mouse Bak by flow cytometry (and immunoprecipitation). When α1 and α2 were tethered (Y41C:A79C) before cells being incubated with Bid, G317-2 bound to the same proportion of cells and with the same efficiency as the untethered samples ( Fig. 5a,b ). Thus, the tethered α1 and α2 helices were able to dissociate as a unit from the rest of the protein to expose the BH4 domain. In contrast, when α1 and α6 were tethered (Α28C:L163C), G317-2 did not bind ( Fig. 5a,b ), indicating that the α1–α6 tether had prevented movement of α1. This is supported by Ab-1 also failing to bind its epitope ( Fig. 5d ), which is located further away from the Α28C:L163C tether ( Supplementary Fig. 4 ). Tethering of WT Bak had an intermediate effect on BH4 exposure, as both G317-2 and Ab-1 binding occurred in the majority of Bid-treated cells ( Fig. 5a,b,d,e ), but less antibody bound to each cell ( Fig. 5c,f ). We interpret the lower mean fluorescence intensity (MFI) to indicate that all Bak molecules changed conformation in response to Bid, but were only partially exposing the G317-2 and Ab-1 epitopes. Thus, the WT tether is less restrictive than the Α28C:L163C tether, and allows sufficient α1 dissociation for some antibody to bind. Notably, when Bak was activated by a Bim BH3 peptide or by heating, BH4 exposure was again restricted by the WT and A28C:L163C tethers ( Supplementary Fig. 5 ), suggesting that α1 dissociation from α6 is a requisite response to all triggers of Bak activation. 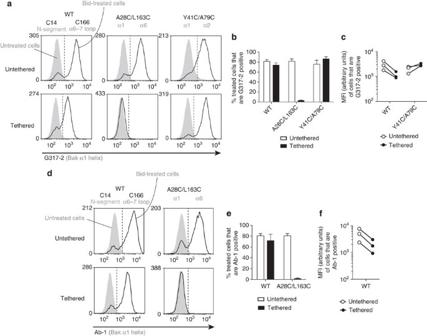Figure 5: Bak BH4 exposure requires dissociation of α1 from α6. (a) Tethering the α1 and α6 helices completely blocks BH4 exposure. Permeabilized DKO MEF expressing Bak (as indicated) were incubated with (tethered) or without (untethered) 200 μM CuPhe, then treated for 30 min with (black lines) or without (filled histograms) 100 nM Bid (30 °C). BH4 exposure was determined by staining with G317-2. Representative FACS plots are shown. (b) Proportion of cells with exposed G317-2 epitope after Bid treatment. The graph shows the percentage cells right of the vertical lines in FACS plots, in Bid-treated samples. Data in graph are mean and s.d. of at least three independent FACS experiments including the data shown ina. (c) Tethering the N-segment to the α6-α7 loop prevents complete G317-2 exposure. Comparison of the mean fluorescent intensities (MFI) of the WT and Y41C/A79C cell populations graphed inb. Lines connect data from the same experiment. (d) Tethering the N terminus to the latch blocks any movement of α1 in response to Bid. Permeabilized DKO MEF expressing WT or A28C/L163C Bak were treated as inaand exposure of an α1 epitope (Ab-1) more distant to the tether than G317-2 (Supplementary Fig. 4) was assessed by FACS. (e) Proportion of cells with exposed Ab-1 epitope after Bid treatment. The graph shows the percentage cells right of the vertical lines in FACS plots, in Bid-treated samples. Data in graph are mean and s.d. of at least three independent FACS experiments including the data shown ind. (f) Tethering the N-segment to the α6–α7 loop prevents complete Ab-1 exposure. Comparison of the mean fluorescent intensities (MFI) of WT cell populations graphed ine. Lines connect data from the same experiment. Figure 5: Bak BH4 exposure requires dissociation of α1 from α6. ( a ) Tethering the α1 and α6 helices completely blocks BH4 exposure. Permeabilized DKO MEF expressing Bak (as indicated) were incubated with (tethered) or without (untethered) 200 μM CuPhe, then treated for 30 min with (black lines) or without (filled histograms) 100 nM Bid (30 °C). BH4 exposure was determined by staining with G317-2. Representative FACS plots are shown. ( b ) Proportion of cells with exposed G317-2 epitope after Bid treatment. The graph shows the percentage cells right of the vertical lines in FACS plots, in Bid-treated samples. Data in graph are mean and s.d. of at least three independent FACS experiments including the data shown in a . ( c ) Tethering the N-segment to the α6-α7 loop prevents complete G317-2 exposure. Comparison of the mean fluorescent intensities (MFI) of the WT and Y41C/A79C cell populations graphed in b . Lines connect data from the same experiment. ( d ) Tethering the N terminus to the latch blocks any movement of α1 in response to Bid. Permeabilized DKO MEF expressing WT or A28C/L163C Bak were treated as in a and exposure of an α1 epitope (Ab-1) more distant to the tether than G317-2 ( Supplementary Fig. 4 ) was assessed by FACS. ( e ) Proportion of cells with exposed Ab-1 epitope after Bid treatment. The graph shows the percentage cells right of the vertical lines in FACS plots, in Bid-treated samples. Data in graph are mean and s.d. of at least three independent FACS experiments including the data shown in d . ( f ) Tethering the N-segment to the α6–α7 loop prevents complete Ab-1 exposure. Comparison of the mean fluorescent intensities (MFI) of WT cell populations graphed in e . Lines connect data from the same experiment. Full size image Full BH4 exposure requires core–latch dissociation Recent studies show that activation of both Bak and Bax requires separation of α5 in the core from α6 in the latch [19] , [20] , raising the possibility that this event occurs before α1 dissociation. For example, the α1–α6 tether in Fig. 5 might be preventing α6 dissociation rather than α1 dissociation. To test the relationship of core–latch separation to α1 dissociation, we utilized the Bak variant V142C/F150C (ref. 20 ). When treated with CuPhe, V142C in α5 was efficiently tethered to F150C in α6 and the tether prevented cytochrome c release in response to Bid [20] . We now show that when V142C/F150C is tethered, binding of both G317-2 and Ab-1 still occurs in the majority of Bid-treated cells ( Fig. 6a, b ), as found for tethered WT Bak ( Fig. 5 ). As binding of Ab-1 would not occur after dissociation of α6–α8 alone ( Supplementary Fig. 3 ), α1 dissociation must be initiated before or in concert with core–latch separation. In addition, as antibody binding is limited in the presence of the tether ( Fig. 6c ), complete α1 dissociation requires α6 dissociation from the core. Altogether, these results indicate that movement of both α1 and the α6-containing latch are required for full exposure of the BH4 domain during activation. 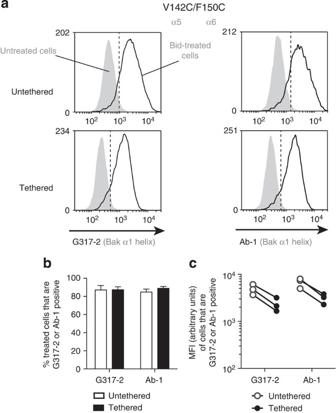Figure 6: Full BH4 exposure requires core–latch dissociation. (a) Dissociation of α1 occurs before or in concert with α6 movement. Permeabilized DKO MEF expressing V142C/F150C Bak were treated with CuPhe and Bid as inFig. 5a. Dissociation of α1 was measured by staining with G317-2 and Ab-1. Representative FACS plots are shown. (b) Proportion of cells with exposed BH4 domain in response to Bid. The graph shows the percentage of cells right of the vertical lines in FACS plots, in Bid-treated samples. Data are mean and s.d. of at least three independent FACS experiments, including the data shown ina. (c) Tethering the core and latch prevents complete BH4 exposure. Comparison of the mean fluorescent intensities (MFI) of V142/CF150C cell populations graphed inb. Lines connect data from the same experiment. Figure 6: Full BH4 exposure requires core–latch dissociation. ( a ) Dissociation of α1 occurs before or in concert with α6 movement. Permeabilized DKO MEF expressing V142C/F150C Bak were treated with CuPhe and Bid as in Fig. 5a . Dissociation of α1 was measured by staining with G317-2 and Ab-1. Representative FACS plots are shown. ( b ) Proportion of cells with exposed BH4 domain in response to Bid. The graph shows the percentage of cells right of the vertical lines in FACS plots, in Bid-treated samples. Data are mean and s.d. of at least three independent FACS experiments, including the data shown in a . ( c ) Tethering the core and latch prevents complete BH4 exposure. Comparison of the mean fluorescent intensities (MFI) of V142/CF150C cell populations graphed in b . Lines connect data from the same experiment. Full size image In addition, we found that another measure of Bak α1 conformation change was cleavage by the serine protease enterokinase (EK). EK cleaved Bak only after it had been activated by Bid, and generated an ∼ 20 kDa membrane-bound fragment ( Supplementary Fig. 6 ). Moreover, the non-canonical cleavage site was within the BH4 domain in α1 as the cleaved fragment was recognized by Ab-1 but not G317-2 ( Fig. 7a ). Notably, cleavage was absent when the N terminus was tethered to the latch (WT, A28CL163C) or the latch was tethered to the core (V142CF150C, Fig. 7b ), indicating that those tethers had blocked BH4 exposure, consistent with our FACS results. Curiously, cleavage was also absent when α1 was tethered to α2 (Y41CA79C, Fig. 7b ) despite full exposure of the G317-2 epitope ( Figs 4d,e and 5a–c ). We suspect the disulfide bond prevents access of EK, but not G317-2, to its target site. These results therefore confirm that movement of both α1- and the α6-containing latch are required for full BH4 exposure during Bak activation. 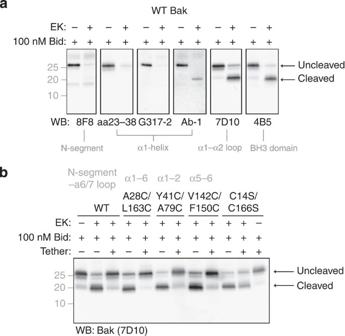Figure 7: Tethering Bak prevents exposure of an enterokinase cleavage site in the BH4 domain. (a) Enterokinase cleaves at the BH4 domain in activated Bak. Permeabilized DKO MEF expressing WT Bak were treated with Bid (+) as inFig. 5a, then incubated for 2 h at room temperature without (−) or with recombinant enterokinase (EK; 3 U per 50 μl). Samples were western blotted with the indicated anti-Bak antibodies. Note that the BH4 domain spans the G317-2 and Ab-1 epitopes (seeFig. 9a). Data are representative of at least two independent experiments. (b) Tethering Bak prevents exposure of enterokinase cleavage site. Permeabilized DKO MEF expressing the indicated Bak variants were treated with CuPhe and Bid as inFig. 5aand with EK as inFig. 7aand then western blotted with the 7D10 antibody as Ab-1 does not bind Y41C/A79C Bak. Note EK was still able to cleave Bid-treated C14S/C166S Bak in the presence of CuPhe. Data are representative of at least two independent experiments. Figure 7: Tethering Bak prevents exposure of an enterokinase cleavage site in the BH4 domain. ( a ) Enterokinase cleaves at the BH4 domain in activated Bak. Permeabilized DKO MEF expressing WT Bak were treated with Bid (+) as in Fig. 5a , then incubated for 2 h at room temperature without (−) or with recombinant enterokinase (EK; 3 U per 50 μl). Samples were western blotted with the indicated anti-Bak antibodies. Note that the BH4 domain spans the G317-2 and Ab-1 epitopes (see Fig. 9a ). Data are representative of at least two independent experiments. ( b ) Tethering Bak prevents exposure of enterokinase cleavage site. Permeabilized DKO MEF expressing the indicated Bak variants were treated with CuPhe and Bid as in Fig. 5a and with EK as in Fig. 7a and then western blotted with the 7D10 antibody as Ab-1 does not bind Y41C/A79C Bak. Note EK was still able to cleave Bid-treated C14S/C166S Bak in the presence of CuPhe. Data are representative of at least two independent experiments. Full size image BH3 exposure is initiated in the absence of BH4 exposure To test whether α2 movement might precede α1 movement, we measured BH3 exposure when α1 was tethered or untethered. It was plausible that BH3 exposure could occur even if α1 was tethered to the protein core due to the length (19 residues) and flexibility of the α1–α2 loop. To capture BH3 exposure, the 4B5 antibody was added during (rather than after) the incubation with Bid, as the BH3 domain is normally only transiently exposed before it binds to another activated Bak molecule [9] . Accordingly, in the untethered samples, 4B5 added during the incubation bound each Bak variant after Bid treatment ( Fig. 8a,b ). Even in the tethered samples, the 4B5 antibody bound to all three Bak variants ( Fig. 8a,b ) indicating that BH3 exposure is a very early step in Bak activation. The α1–α6 tether (A28C:L163C) was most informative as it fully blocked BH4 exposure ( Fig. 5 ) but not BH3 exposure ( Fig. 8a,b ). Thus, when Bid binds to the Bak hydrophobic groove, BH3 exposure is initiated before BH4 exposure. 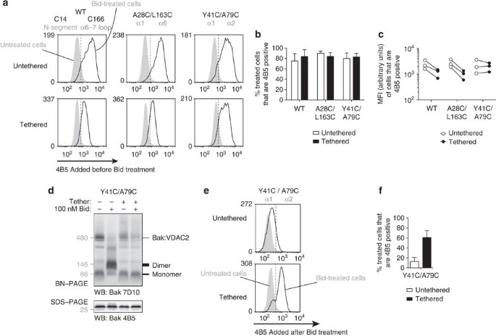Figure 8: Bak BH3 exposure precedes BH4 exposure, but dimerization requires dissociation of α1 from α2. (a) Tethering of the N terminus to α2 or the α6–α8 latch allows BH3 exposure. Permeabilized DKO MEF expressing Bak (as indicated) were treated with CuPhe and Bid as inFig. 5a. BH3 exposure was detected by the addition of 4B5 to cells before Bid, because the 4B5 epitope is part of the BH3:groove interface9and thus inaccessible after Bid treatment. Representative FACS plots are shown. (b) Proportion of cells with an exposed BH3 domain in response to Bid. The graph shows the percentage of cells, right of the vertical lines in the plots, in Bid-treated samples. Data are mean and s.d. of at least three independent FACS experiments, including the data shown ina. (c) The N-segment and α1 must dissociate from the α6–α8 latch for complete BH3 exposure. Comparison of mean fluorescent intensities (MFIs) of cell populations graphed inb. Lines connect data from the same experiment. (d) Tethering α1 to α2 prevents BH3:groove dimerization. Permeabilized DKO MEF expressing Y41C/A79C Bak were treated with CuPhe and Bid as inFig. 5a. Bak dimers and monomers were resolved by Blue Native (BN)–PAGE and visualized after western blot. SDS–PAGE of samples indicated equivalent loading. Data are representative of two independent experiments. (e) Tethering α1 to α2 results in persistent exposure of BH3 domains in response to Bid. Permeabilized DKO MEF expressing Y41C/A79C Bak were treated with CuPhe and Bid as inFig. 5aand subsequently incubated with 4B5. Representative FACS plots are shown. (f) Proportion of cells with BH3 domains exposed after responding to Bid, indicating an inability to form homodimers. The graph shows the percentage of cells right of the vertical line, after Bid treatment. Data in graph are mean and s.d. of at least three independent FACS experiments, including the data shown ine. Figure 8: Bak BH3 exposure precedes BH4 exposure, but dimerization requires dissociation of α1 from α2. ( a ) Tethering of the N terminus to α2 or the α6–α8 latch allows BH3 exposure. Permeabilized DKO MEF expressing Bak (as indicated) were treated with CuPhe and Bid as in Fig. 5a . BH3 exposure was detected by the addition of 4B5 to cells before Bid, because the 4B5 epitope is part of the BH3:groove interface [9] and thus inaccessible after Bid treatment. Representative FACS plots are shown. ( b ) Proportion of cells with an exposed BH3 domain in response to Bid. The graph shows the percentage of cells, right of the vertical lines in the plots, in Bid-treated samples. Data are mean and s.d. of at least three independent FACS experiments, including the data shown in a . ( c ) The N-segment and α1 must dissociate from the α6–α8 latch for complete BH3 exposure. Comparison of mean fluorescent intensities (MFIs) of cell populations graphed in b . Lines connect data from the same experiment. ( d ) Tethering α1 to α2 prevents BH3:groove dimerization. Permeabilized DKO MEF expressing Y41C/A79C Bak were treated with CuPhe and Bid as in Fig. 5a . Bak dimers and monomers were resolved by Blue Native (BN)–PAGE and visualized after western blot. SDS–PAGE of samples indicated equivalent loading. Data are representative of two independent experiments. ( e ) Tethering α1 to α2 results in persistent exposure of BH3 domains in response to Bid. Permeabilized DKO MEF expressing Y41C/A79C Bak were treated with CuPhe and Bid as in Fig. 5a and subsequently incubated with 4B5. Representative FACS plots are shown. ( f ) Proportion of cells with BH3 domains exposed after responding to Bid, indicating an inability to form homodimers. The graph shows the percentage of cells right of the vertical line, after Bid treatment. Data in graph are mean and s.d. of at least three independent FACS experiments, including the data shown in e . Full size image We also noted that 4B5 binding was limited in tethered WT and Α28C/L163C, as shown by lower MFI after tethering ( Fig. 8c ). This limited 4B5 binding suggests that flexion of the α1–α2 loop is not sufficient for complete BH3 exposure. Instead, α1 dissociation from the α6–α8 latch domain is also required, as suggested by complete BH3 exposure when α1 was tethered to α2 (Y41C:A79C, Fig. 8a–c ). Dimer formation requires dissociation of α1 from α2 We noted that one tether (Y41C:A79C) allowed Bid treatment to expose both the BH4 and BH3 domains ( Figs 5a,b and 7a,b ) but did not allow cytochrome c release ( Fig. 4c ). As α1 was still linked to α2, the exposed BH3 domain may have been unable to bind the hydrophobic groove of another activated Bak molecule to form a BH3:groove homodimer. This was confirmed by Blue-Native–PAGE experiments in which tethered Bak Y41C/A79C failed to dimerize following Bid treatment ( Fig. 8d ). In addition, the BH3 domain remained exposed as shown by 4B5 antibody binding after (rather than during) the Bid incubation ( Fig. 8e,f ). Thus, Bak α1 must dissociate from α2 for Bak dimerization and pore formation. In summary, Bak activation by Bid, Bim or heat proceeds via movement of α2 followed by dissociation of α1 from both the α2–α5 core domain and the α6–α8 latch domain. Separation of the latch from core does not occur before α1 dissociation, but may occur in concert as contacts between helices are progressively lost. The resulting exposure of hydrophobic residues in multiple helices may drive further conformation changes that promote Bak oligomerization due to the newly exposed residues engaging in new protein–protein or protein–lipid interactions. To delineate the Bak ‘N-terminal conformation change’ known for many years to occur during apoptosis, we mapped N-terminal epitopes (summarized in Fig. 9a ) and assayed their exposure in combination with disulfide tethering ( Figs 4 , 5 , 6 , 7 , 8 ). Our data show that during apoptosis, the N-segment and α1 of Bak dissociate entirely from the rest of the protein to expose the BH4 domain and other residues ( Fig. 9b ), consistent with recent reports that Bak α1 and α6 became >50 Å apart after tBid treatment in LUV [26] and the distance between Bax α1 and α2 varies widely after activation [21] . Disulfide tethering of Bak showed that α1 dissociation from both the core (α2–α5) and the latch (α6–α8) was required for pore formation. Furthermore, our novel approach of combining tethers with FACS analysis of epitope exposure suggested that Bak conformation change initiates with movement of α2, followed by α1 dissociation, and that both events are required for complete BH3 exposure and subsequent dimerization. 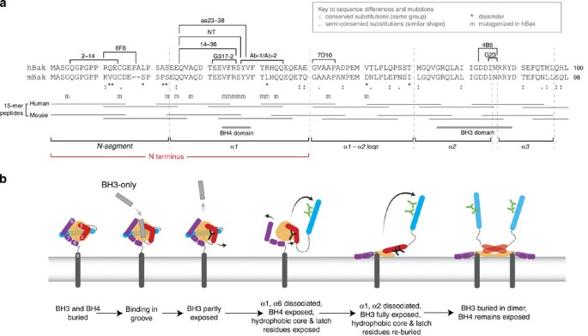Figure 9: Summary of epitope mapping data and sequence of conformation changes during Bak activation. (a) Diagram showing the position of Bak antibody epitopes, 15-mer peptides (mouse and human), amino acid differences, mutagenized residues and structural and functional domains in the first 100 residues of Bak. (b) Diagram showing the sequence of conformation changes that Bak undergoes during activation. The α1 (blue), core (orange/red), latch domain (purple) and transmembrane domain (dark grey) are illustrated.Yindicates an epitope is partially accessible to antibody, that is, 4B5 in black, or G317-2 or Ab-1 in green.YYindicates an epitope is fully accessible to antibody. Bak activation is initiated by transient binding of BH3-only domains to the hydrophobic groove, provoking movement of α2 and BH3 exposure. Movement of α2 also breaks α1 contact with the α6–α8 latch, leading to exposure of the BH4 domain and hydrophobic and aromatic residues in the core and latch domains. Dissociation of α1 from the latch allows α2 to reach a position where the BH3 domain is fully exposed. Consequently, exposed hydrophobic and aromatic residues in the core and latch become buried in the membrane, or in interactions with other helices to promote formation of symmetric dimers. Figure 9: Summary of epitope mapping data and sequence of conformation changes during Bak activation. ( a ) Diagram showing the position of Bak antibody epitopes, 15-mer peptides (mouse and human), amino acid differences, mutagenized residues and structural and functional domains in the first 100 residues of Bak. ( b ) Diagram showing the sequence of conformation changes that Bak undergoes during activation. The α1 (blue), core (orange/red), latch domain (purple) and transmembrane domain (dark grey) are illustrated. Y indicates an epitope is partially accessible to antibody, that is, 4B5 in black, or G317-2 or Ab-1 in green. YY indicates an epitope is fully accessible to antibody. Bak activation is initiated by transient binding of BH3-only domains to the hydrophobic groove, provoking movement of α2 and BH3 exposure. Movement of α2 also breaks α1 contact with the α6–α8 latch, leading to exposure of the BH4 domain and hydrophobic and aromatic residues in the core and latch domains. Dissociation of α1 from the latch allows α2 to reach a position where the BH3 domain is fully exposed. Consequently, exposed hydrophobic and aromatic residues in the core and latch become buried in the membrane, or in interactions with other helices to promote formation of symmetric dimers. Full size image The requirement of α1 dissociation for Bak function is consistent with the role of α1, and more specifically the BH4 domain, in stabilizing the non-activated conformation of Bak. The BH4 motif is highly conserved in multidomain Bcl-2 proteins including viral prosurvival proteins [15] . Its role in stabilizing Bak is indicated by the structure of non-activated Bak in which the four hydrophobic residues in the BH4 domain ( 34 VFxxYV 39 ) contact four neighbouring helices (α2, α5, α6, α7) [3] . R42 may also stabilize non-activated Bak, as structurally this residue participates in a hydrogen bond network with α3 (ref. 3 ). As α1 makes many contacts with other helices, α1 dissociation may be triggered by disrupting one or more of those contacts. A recent crystal structure of Bim peptide bound to the Bax groove demonstrated α2 movement, and formation of a cavity between helices 2, 5 and 8 (ref. 19 ). An NMR structure of Bid peptide bound to the Bak groove also indicated perturbations in several helices including α1, α2 and α6 (ref. 12 ). The present studies show α2 movement as a very early consequence of Bid binding to the Bak groove. Thus, α2/3 movement and cavity formation may individually or in concert trigger α1 dissociation. Dissociation of α1 allows Bak to unfold into three major components: the N terminus, the core (α2–α5) and the latch (α6–α8). This unfolding exposes many hydrophobic residues in α1, α2 and α5–α8 ( Supplementary Fig. 7 ) that engage in new protein–lipid or protein–protein interactions to porate the MOM. For example, recent structural and biochemical studies indicate that protein–lipid interactions occur as Bak collapses onto the membrane, with α4, α5 and α6 lying in-plane on the MOM surface [19] , [26] . The amphipathic α7 and α8 may also lie in-plane to protect their hydrophobic and aromatic residues. Protein–protein interaction generates dimers when the exposed BH3 domain in α2 binds to the hydrophobic groove of another Bak molecule [9] , [22] . In contrast, α1 remains solvent-exposed as all epitopes can be bound by antibodies in immunoprecipitation or intracellular FACS assays, including those that involve hydrophobic regions such as the BH4 domain. Solvent-exposure of the N terminus is consistent with increased susceptibility of activated Bak to proteolysis by proteinase K, trypsin, calpain [11] , [27] , [28] , [29] and enterokinase ( Fig. 7 ). Thus, unlike the core and latch domains, the N terminus does not participate in forming the apoptotic pore, consistent with the ability of N-terminally truncated Bak or Bax to permeabilize mitochondria [14] , [30] . Dissociation of α1 may also be necessary for heterodimerization with the prosurvival proteins Bcl-x L and Mcl-1, as heterodimers form via a BH3:groove interaction [27] , [31] . Dissociation of α1 before heterodimerization is consistent with exposure of a calpain cleavage site at R42 in α1 in the Bak:Bcl-x L complex [27] , and even with interaction of the Bax α1 with α1 of Bcl-x L (ref. 32 ). Where Bcl-x L has apparently prevented exposure of N-terminal epitopes in Bak or Bax (as measured by immunoprecipitation assays) [17] , [25] , [27] , it is likely that Bcl-x L prevented Bak/Bax activation via Mode 1 interactions with BH3-only proteins [27] or that it masked the Bak or Bax epitopes. Three factors hint that α1 may not retain the helical conformation evident in the structure of non-activated Bak [3] . First, all epitopes in α1 appear linear based on their binding to Bak after SDS–PAGE and to the peptide array. Second, calpain cleaves activated Bak at R42/H43 toward the end of α1 (ref. 12 ), and calpain rarely cleaves in helical regions [33] . Third, if α1 did remain helical, the hydrophobic surface (for example, the BH4 domain) that normally faces the hydrophobic core of Bak might be expected to make further protein–protein or protein–lipid interactions. But instead, all regions remain available for antibody binding. Like Bak, Bax N-terminal epitopes (for the 6A7, Bax NT and Bax N20 antibodies) become exposed following apoptosis. Moreover, the epitopes are in the region of Bax α1 (residues 13–19, 1–21 and 11–30, respectively) that abuts the α6–α8 latch domain [34] , [35] , [36] , and the epitopes of polyclonal Bax N20 may even include residues of the Bax BH4 domain ( 26 LLQGFI 31 ). As Bax N-terminal exposure is akin to that for Bak, α1 dissociation is probably also required for Bax activation and pore formation. Indeed, tethering the Bax α1–α2 loop to α6 blocked 6A7 exposure and cytochrome c release in response to SAHB Bim peptide [37] . In this case, the binding site was the ‘rear pocket’ formed by Bax α1/α6, suggesting that α1 dissociation is a key event in Bax and Bak activation regardless of the initiating interaction. In conclusion, detailed characterization of the epitopes of several commonly used Bak antibodies, together with a novel tethering approach, enabled us to determine that α1 dissociation is a crucial step in Bak (and probably Bax) activation. With the restraining influence of α1 removed, the freed core and latch domains are able to orient in the membrane, enabling dimerization, oligomerization, cytochrome c release and ultimately cell destruction. Thus, interference with α2 movement or α1 dissociation may represent a new strategy for therapeutic intervention in pathologies associated with overactive or inefficient Bak-mediated apoptosis. Antibodies and other materials Anti-Bak antibodies were obtained from suppliers and diluted as indicated in Table 1 . Other primary antibodies used were anti-cytochrome c (Clone 7H8.2C12, 1:1,000, BD #556433) and anti β-actin (Clone AC-15, 1:20,000, Sigma #A1978). Secondary antibodies used for western blotting were horseradish peroxidase (HRP)-conjugated sheep anti-mouse (1:2,000, Amersham #NXΑ931), goat anti-rabbit (1:5,000, Southern Biotech #4010-05) and goat anti-rat (1:5,000, Southern Biotech #3010-05) IgGs. To avoid nonspecific signals from the light chains of IP antibodies, which are very similar in size to Bak, FC ϒ chain-specific HRP-conjugated goat anti-rat IgG (1:5,000, Southern Biotech #3030-05) was used for IP western blots ( Figs 3 and 4d ). Secondary antibodies used for FACS were RPE-labelled goat anti-rat (1:200, Southern Biotech #3050-09) or goat anti-mouse (1:200, Southern Biotech #1031-09) IgGs. Bim BH3 peptide [38] (H-DMRPEIWIAQELRRIGDEFNAYYARR-NH2) was synthesized by Mimotopes, reconstituted in dimethyl sulfoxide (10 mM) and kept at −20 °C. Redox catalyst copper(II)(1,10-phenoanthroline) 3 (CuPhe) stocks were prepared with 30 mM CuSO 4 and 100 mM 1,10-phenoanthroline in 4:1 water:ethanol and stored at −20 °C. Cell culture Phoenix cells, DU145 and SV40-transformed mouse embryonic fibroblasts derived from Bak −/− Bax −/− mice (DKO MEF) and Bax −/− mice were a gift from Professor David Huang. Note, the DU145 cells were obtained from the Frederick National Laboratory (USA) as part of the NCI-60 panel of cell lines [39] . DKO MEF, DKO MEF expressing Bak variants (see below), Bax −/− MEF and Phoenix cells were maintained in Dulbecco’s modified Eagle’s medium (DMEM) supplemented with 10% fetal calf serum (FCS), 250 μM L-asparagine and 55 μM 2-mercaptoethanol. DU145 cells were maintained in DMEM supplemented with 10% FCS. All lines were routinely passaged by rinsing cells with phosphate-buffered saline (PBS) and incubating with trypsin for 3–10 min, and then resuspending cells (diluted 1:2 to 1:30) in fresh medium. All lines were cultured at 37 °C in 10% CO 2 . Site-directed mutagenesis Cysteine variants and N-terminal truncations of Bak were generated by cloning the product of three sequential PCRs (see below) into the pMX-IG vector, kindly provided by Professor David Huang. Primers ( Supplementary Table 1 ) were purchased from GeneWorks Pty Ltd. For each mutation (except the truncations), two initial paired reactions were performed. One reaction contained the relevant internal (mutagenic) forward primer and a Bak reverse primer that includes an XhoI site. The second reaction contained an hBak forward primer that includes an EcoRI site and the matching internal (mutagenic) reverse primer. Each reaction mixture contained 20 ng template DNA, 0.5 μM of each primer and 1 × Phusion PCR Master Mix (Finnzymes, #F-531S) and were incubated in an MJ Research PTC-200 Thermal Cycler or a Bio-Rad T100 Thermal Cycler. Cycling conditions were: 94 °C, 2 min; 30 cycles of (94 °C, 35 s; 58 °C, 30 s; 72 °C, 60 s); 72 °C, 5 min. The two resulting complementary DNA fragments were gel-purified using the Wizard SV Gel and PCR Cleanup kit (Promega, #A9282) and each pair of DNAs (3 μl each) annealed by incubation with 1 × Phusion PCR Master Mix in a total volume of 25 μl. The incubation conditions were: 10 cycles of (94 °C, 35 s; 65 °C, 30 s; 72 °C, 60 s). The annealed DNAs were then amplified using the hBak forward and reverse primers. Reaction mixtures contained 3 μl annealed DNA, 0.5 μM of each primer and 1 × Phusion PCR Master Mix in a total volume of 50 μl. The cycling conditions were: 94 °C, 2 min; 25 cycles of (94 °C, 35 s; 58 °C, 30 s; 72 °C, 60 s); 72 °C, 5 min. Gel-purified reaction products and the pMX-IG vector were digested overnight at 37 °C with the EcoRI and XhoI restriction enzymes (Roche, #10703737001 and #10899194001) in SuRE/Cut Buffer H (Roche, #11417991001). Gel-purified digested mutant Bak and vector DNAs (1:3 vector:insert ratio) were incubated overnight at room temperature in 1 × ligase buffer containing 2U T4 DNA ligase (Promega, #M1801). Ligation products were used to transform electro-competent JM109 cells and colonies grown overnight on LB agar plates supplemented with 100 μg ml −1 ampicillin. Subclones were picked, grown overnight and their DNA purified using a QIAprep Spin Mini Kit (QIAGEN, #27106) and stored at −20 °C. Positive clones were identified by restriction digestion, confirmed by sequencing and used for retroviral transfection. Retroviral transfection and transduction Bak variants were stably expressed in DKO MEF by retroviral infection. pMX-IG constructs were transfected into Phoenix cells using FuGENE6 (Promega, #E2691) or X-tremeGENE 9 (Roche, #06365787001) according to the manufacturers’ instructions. DKO MEF at 70–80% confluency in six-well tissue culture plates were transduced with filtered (0.45 μM) viral supernatants ( ∼ 4 ml each) mixed with 4 μg ml −1 polybrene (Sigma, #107689-10G). After centrifugation (1,083 g , 45 min, 32 °C), cells were incubated for 24 h, the viral supernatants replaced with fresh media and cells passaged. After a further 24–48 h at 37 °C, cells were resuspended in buffer (10% FCS: 90% (150 mM NaCl, 3.7 mM KCl, 2.5 mM CaCl 2 , 1.2 mM MgSO 4 , 14.8 mM HEPES)), filtered and polyclonal GFP-positive populations isolated by FACS using a MoFlo Legacy machine (Beckman Coulter). To prevent infection, sorted cells were cultured in media containing ciprofloxacin (Bayer) for the first 2 weeks. Peptide scanning arrays Three sets of N-terminally biotinylated Bak peptides (with SGSG linker sequence) were synthesized by Mimotopes: (i) 21 15-mer, with a five-residue overlap, spanning all residues of mouse Bak; (ii) 21 15-mer, with a five-residue overlap, spanning all residues of human Bak; (iii) 39 8-mer, with a one-residue offset, spanning residues 20–65 of human Bak. Each lyophilized peptide (1–3 mg each) was resuspended in 400 μl 80% dimethylformamide (DMF) and stored at −80 °C. 96-well plates (Nunc Immuno Maxisorp, #442404 or Corning Costar non-treated PVC, #2797) were coated with 5 μg ml −1 streptavidin (Sigma S-4762) by incubation for 16–24 h at 37 °C. Plates were washed four times with PBS-T (0.1% Tween 20 in PBS), blocked by incubating for 1 h at ∼ 21 °C in PBS-T containing 0.5% (w/v) BSA (Sigma) and again washed four times in PBS-T. Peptides (in DMF) were diluted 1:1,000 with H 2 O and 100 μl each added to wells of prepared plates. After 1 h incubation, with shaking, unbound peptides were removed by washing four times with PBS-T. Primary antibodies were diluted (see Table 1 ) in PBS-T and 100 μl incubated with each peptide for at 1 h at room temperature on a rocking platform. Plates were washed four times with PBS-T and 100 μl HRP-conjugated secondary antibody, diluted with PBS-T, was added and plates incubated at room temperature for 1 h on a rocking platform. Dilutions of secondary antibodies were as for western blots, except for peptide set (iii) where the anti-rabbit and anti-rat antibodies were diluted 1:10,000. Plates were washed four times with PBS-T and bound secondary antibody was detected by incubating with 100 μl ABTS buffer (1 mM ABTS (2,2′-Azino-bis(3-ethylbenzthiazoline-6-sulfonic acid)) diammonium salt, Sigma, #Α1888), 100 mM citric acid, 0.03% H 2 O 2 ) for 10–45 min and measuring absorbance at 405 nM using a Hidex Chameleon V Multitechnology Platereader. Bak tethering and activation MEF were harvested with trypsin, washed with PBS and the outer cell membrane permeabilized by resuspending cells at 1 × 10 7 ml −1 in ice-cold MELB buffer (20 mM HEPES/NaOH pH 7.5, 100 mM sucrose, 2.5 mM MgCl 2 , 100 mM KCl, 1 × complete protease inhibitor (Roche), 4 μg ml −1 pepstatin A) containing 0.025% digitonin. After 5 min incubation on ice, cell permeabilization was verified by uptake of trypan blue. For cytochrome c release assays and IPs, permeabilized cells were centrifuged (16,200 g , 5 min, 4 °C) and membrane fractions resuspended in MELB buffer and kept on ice. For enterokinase cleavage assays of Bak, membrane fractions were permeabilized and subsequently resuspended in MELB buffer lacking 1 × complete protease inhibitor. Intramolecular tethers were induced by disulfide bonding of cysteines using CuPhe diluted 500-fold into the sample. Permeabilized MEF or membrane fractions were incubated with CuPhe at least 5 min on ice. The efficiency of tethering was assessed by western blotting after mixing untreated or CuPhe-treated samples with an equal volume of sample buffer (0.15 M Tris pH 6.8, 30% glycerol, 1.2% SDS, 0.018 mg ml −1 bromophenol blue) containing 25 mM EDTA to chelate the copper. To induce Bak activation, untreated or CuPhe-treated samples were incubated with 100 nM caspase-8 cleaved human Bid or 10 μM Bim BH3 peptide for 30 min at 30 °C, or for 30 min at 44 °C. Activation reactions were stopped by placing samples on ice for at least 5 min. Cytochrome c release Following activation of Bak in membrane fractions, the samples were centrifuged at 16,200 g , 5 min, 4 °C. The resulting supernatant and pellet fractions were each mixed with sample buffer containing 5% (v/v) 2-mercaptoethanol (2Me) and western blotting performed for cytochrome c . Immunoprecipitation of activated Bak Following activation of Bak in membrane fractions, samples were solubilized by incubation with 1% digitonin on ice for at least 30 min. Samples were centrifuged (16,200 g , 5 min, 4 °C) and supernatants pre-cleared by 30 min incubation at 4 °C with Protein G Sepharose beads 4 Fast Flow (GE Healthcare Life Sciences), pre-washed with Onyx buffer (20 mM TrisCl pH 7.4, 135 mM NaCl, 1.5 mM MgCl 2 , 1 mM EGTA, 10% glycerol, 1 × complete protease inhibitor, 4 μg ml −1 pepstatin A). After removing beads by repeated washes in Onyx buffer, lysates were incubated with constant agitation for 2 h at 4 °C with 4 μg ml −1 anti-Bak antibody, followed by incubation for 1 h at 4 °C with additional pre-washed Sepharose G beads. Immune complexes were isolated by centrifugation (16,200 g , 2 min, 4 °C), washed four times with Onyx buffer, resuspended in sample buffer containing 5% (v/v) 2Me and analysed by western blotting. FACS analysis Following activation of Bak in permeabilized cells, the samples were centrifuged (900 g , 3 min, 4 °C), cells were washed with FACS buffer (10% FBS: 90% (1.2 mM MgSO 4 , 7.4 mM HEPES-NaOH, 0.8 mM K 2 HPO 4 , 140 mM NaCl)) and incubated 40–70 min on ice with anti-Bak antibodies (Ab-1, G317-2 or 4B5) diluted 1:100 in FACS buffer. To assess BH3 domain exposure during Bak activation, 10 μg ml −1 anti-Bak (4B5) antibody was added to untreated and CuPhe-treated samples immediately before the Bak activation step. After incubation with primary antibody, cells were washed with FACS buffer and incubated 40–70 min on ice with RPE-labelled secondary antibody diluted 1:200 in FACS buffer. The cells were washed with FACS buffer and data collected immediately using an LSRII flow cytometer (BD) fitted with FACSDiVa software (BD) were subsequently analysed using WEASEL (v2.7). Doublets and debris were routinely excluded by gating using forward scatter cytometry and side scatter cytometry. To quantify the proportions of cells with exposed BH4 or BH3 domains, a marker was positioned to distinguish negatively and positively staining populations, with untreated cells (grey histograms) used as guides for negative staining. The MFI of cells in positive-staining populations was also compared in cases where the proportions of cells appeared similar but the amount of staining (that is, profile position on x axis) differed in tethered versus untethered cells. Bak cleavage by EK Following tethering and/or activation of Bak in membrane fractions, samples were incubated with or without recombinant EK (3 or 4.4 units per 50 μl sample; Merck #69066-3) for 2 h at room temperature. EK was inactivated by the addition of PMSF (4 mM) and cleavage assessed by western blotting after mixing samples with an equal volume of sample buffer containing 5% (v/v) 2Me. Blue Native–PAGE Blue Native–PAGE was performed after Bak activation in permeabilized MEF (as described above) using the Invitrogen NativePAGE Novex Bis-Tris Gel System. All samples were incubated 30 min on ice, centrifuged (16,200 g , 5 min, 4 °C) and the pellets resuspended in Solubilization buffer (20 mM Bis-Tris pH 7.4, 50 mM NaCl, 10% glycerol, 1% digitonin). After at least 30 min on ice, the samples were centrifuged (16,200 g , 5 min, 4 °C), the supernatants mixed with NativePAGE sample buffer and NativePAGE 5% G-250 sample additive and proteins separated on 4–16% NativePAGE Novex Bis-Tris gels in chambers containing 1 × NativePAGE anode buffer and 1 × NativePAGE cathode buffer containing 1 × NativePAGE cathode additive. After running at 150 V for 30–45 min, the blue cathode buffer was replaced with 1 × NativePAGE cathode buffer without any cathode additive and gels run for a further 80–95 min. Proteins were transferred to polyvinylidene difluoride membranes at 40 V for 150 min in buffer containing 25 mM Tris, 192 mM glycine, 20% methanol and 0.037% SDS. Membranes were de-stained by ∼ 40 min incubation in fixative [10% acetic acid, 45% methanol]. After washing 3 times for 10 min in water, membranes were incubated in blocking solution and proteins detected by Western blotting. To compare sample loading, excess sample was mixed 1:1 with sample buffer containing 5% (v/v) 2Me and analysed by western blotting. Western blotting Samples were heated 5 min at >95 °C, spun briefly and proteins separated by SDS–PAGE using pre-cast 12% TGX gels (Bio-Rad) and transferred to nitrocellulose membranes at 40 V for 150 min in buffer containing 25 mM Tris, 192 mM glycine and 20% methanol. Note that transfer of proteins to polyvinylidene difluoride rather than nitrocellulose membranes resulted in inferior signals for most Bak antibodies (data not shown). Nonspecific binding of antibodies was blocked by incubation for 30–45 min with 5% nonfat milk powder in TBS (20 mM TrisHCl pH7.6, 137 mM NaCl) with 0.1% Tween 20. Membranes were rinsed with TBS/0.1% Tween 20 and incubated with primary antibodies at room temperature for 1–5 h or at 4 °C overnight. The Ab-1, Ab-2 and 4B5 anti-Bak antibodies and anti-cytochrome c antibody were diluted in TBS/0.05% Tween 20, anti-β-actin antibody was diluted in TBS/5% BSA. All other primary antibodies were diluted in blocking solution. Membranes were washed three times (5 min each) in TBS/0.1% Tween 20 and incubated 1–2 h at room temperature with secondary antibody diluted in blocking solution, except for cytochrome c blots where the anti-mouse secondary was also diluted in TBS/0.05% Tween 20. Membranes were washed three times (5 min each) in TBS/0.1% Tween 20, developed with Luminata Forte HRP substrate (Millipore) and bioluminescent signals detected using a ChemiDoc XRS+ System fitted with ImageLab software (Bio-Rad). Uncropped images from Figs 1 , 2 , 3 , 4 , 7 and 8 are shown in Supplementary Figs 8–12 . Structural modelling The inactive Bak structure 2IMS 3 was downloaded from PDB and manipulated using PyMOL (DeLano Scientific LLC). The images were saved as PNG files. How to cite this article: Alsop, A. E. et al. Dissociation of Bak α1 helix from the core and latch domains is required for apoptosis. Nat. Commun. 6:6841 doi: 10.1038/ncomms7841 (2015).